Spin–orbit induced electronic spin separation in semiconductor nanostructures The demonstration of quantized spin splitting by Stern and Gerlach is one of the most important experiments in modern physics. Their discovery was the precursor of recent developments in spin-based technologies. Although electrical spin separation of charged particles is fundamental in spintronics, in non-uniform magnetic fields it has been difficult to separate the spin states of charged particles due to the Lorentz force, as well as to the insufficient and uncontrollable field gradients. Here we demonstrate electronic spin separation in a semiconductor nanostructure. To avoid the Lorentz force, which is inevitably induced when an external magnetic field is applied, we utilized the effective non-uniform magnetic field which originates from the Rashba spin–orbit interaction in an InGaAs-based heterostructure. Using a Stern–Gerlach-inspired mechanism, together with a quantum point contact, we obtained field gradients of 10 8 T m −1 resulting in a highly polarized spin current. In 1922, Stern and Gerlach [1] , [2] demonstrated the quantization of spin angular momentum by showing the spatial separation of deflected, uncharged silver particles under an inhomogeneous magnetic field in the experiment named after them. Spin-up and spin-down angular momenta were accelerated in opposite directions due to the spatial modulation of the Zeeman field. However, when applied to charged particles, such as electrons, an additional force, known as the Lorentz force, modulates their orbital motion and hampers the spin separation of the electrons. Therefore, the application of the Stern–Gerlach experiment has been limited to atomic beams [3] , [4] and to propagated light [5] , [6] , as their particles are uncharged. In a two-dimensional system, although the electron orbital motion is restricted in-plane due to the strong potential confinement, external magnetic fields or micromagnets produce either insufficient or uncontrollable field gradients, which make it difficult to separate electron spin. More recent developments in spintronics, where the spin degree of freedom is used for additional information storage, depend heavily on the ability to generate an electron spin flow (spin current) in electric devices. The spin Hall effect provides a method for generating spin current in semiconductors [7] , [8] , [9] . The efficiency of the spin current generation is represented by the spin Hall angle γ SHE , the ratio between a longitudinal conductivity and the spin Hall conductivity. Typically, the spin Hall angle for conventional semiconductor materials is 0.0001 (ref. 10 ), which is too small for use in spintronic devices. Although the spin Hall effect originates from the spin-dependent force induced by the spin–orbit interaction (SOI), spin separation by the spatial modulation of SOI [11] , [12] , [13] has yet to be demonstrated. As the Rashba SOI [14] strength α is tuned by the external-gate electric field [15] , [16] , a non-uniform SOI system can be achieved using the Rashba SOI. When the strength of the Rashba SOI depends on the y direction, α ( y ), the effective force is represented as where σ is the Pauli spin matrix and k x is the conduction electron momentum in the x direction. This force is represented by the 2×2 matrix acting on the SU(2) spin space and results in spin separation in the y direction when electrons are propagated in the x direction. In the original Stern–Gerlach experiment, a metre scale apparatus was necessary to provide for the clear separation of up and down spins due to the small magnetic field gradient of the order of 10 3 –10 4 T m −1 . The effective magnetic field induced by the Rashba SOI is much larger, at more than 10 T on the nanometre scale [17] . By spatially modulating the effective magnetic field with a field effect transistor structure, the spin-dependent force can be enhanced considerably. Here we demonstrate an experimental manifestation of electronic Stern–Gerlach spin separation by using the Rashba SOI in InGaAsP/InGaAs-based field effect transistors. The non-uniform Rashba SOI is realized by the lateral potential confinement by the side gate, known as the quantum point contact (QPC) [18] , [19] . The spin-dependent deflection angle γ SGE defined by the ratio between the velocity in the x direction and spin-dependent velocity in the y direction is as large as 0.65, which is significantly larger than the spin Hall effect. We show that the non-uniform SOI induces spin-dependent deflection before the electron is transmitted through the QPC constriction, as is the case in the Stern–Gerlach spin separation, and the scattering due to the potential of the QPC constriction results in spin-dependent transmission/reflection, which in effect produces a spin-polarized electric current. As a result of the spin separation, a spin-resolved plateau with a half integer in units of 2 e 2 / h appears. We have found that the spin polarization of the conduction electrons in this plateau is as high as 70%. Our new approach to generating spin polarization in semiconductor nanostructures provides a way to seamlessly integrate electrical spin generation, manipulation and detection in a single semiconductor device without the need for either external magnetic fields or magnetic materials. Theory of the electronic Stern–Gerlach spin separation The central idea of this study is to combine a strong Rashba SOI system with a QPC to induce spatial modulation of the effective magnetic field. A spin-dependent force is generated by the lateral potential confinement, which separates the spin-up and -down electrons, and the selective filtering of the spin components at the QPC potential results in a spin-split single channel as schematically shown in Fig. 1 . Channel conductance is controlled by the trench-type side gates shown in the s.e.m. image in Fig. 1 . 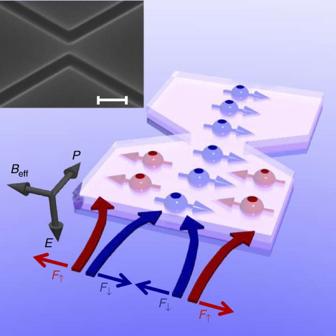Figure 1: Stern–Gerlach type spin separation in a QPC structure. The device comprises an InGaAs/InGaAsP two-dimensional electron gas with strong Rashba SOI. Black arrows correspond to the directions of the electron momentumP, the internal electric fieldEand the effective magnetic fieldBeff. Thin red and blue arrows labelledF↑andF↓are the directions of the spin-dependent force for up and down spins. Thick red and blue arrows are the deflected electron trajectories, and the direction of the electron spin is indicated by blue and red, respectively. The inset shows an image of a QPC channel region taken by a scanning electron microscope. Scale bar=1 μm. Figure 1: Stern–Gerlach type spin separation in a QPC structure. The device comprises an InGaAs/InGaAsP two-dimensional electron gas with strong Rashba SOI. Black arrows correspond to the directions of the electron momentum P , the internal electric field E and the effective magnetic field B eff . Thin red and blue arrows labelled F ↑ and F ↓ are the directions of the spin-dependent force for up and down spins. Thick red and blue arrows are the deflected electron trajectories, and the direction of the electron spin is indicated by blue and red, respectively. The inset shows an image of a QPC channel region taken by a scanning electron microscope. Scale bar=1 μm. Full size image For a detailed exploration of the spin-separation mechanism owing to the Rashba SOI, we calculate the spin polarization in the QPC by employing wave-packet dynamics (for detailed calculations, see Supplementary Methods ). We consider the saddle point potential for the QPC potential landscape and take into account the spatial modulation of the Rashba SOI. 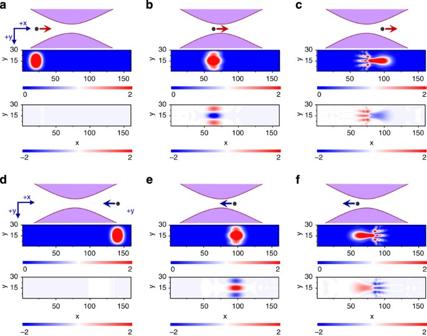Figure 2: Time evolution of the wave packet for the charge density and the spin density in the QPC channel. The three panels ina–findicate the position of the electron wave packet, the charge density and the spin density in the QPC device. Colour bars beneath the panels correspond to scales of charge density between 0 and 2×10−3, and spin density between −2×10−3and +2×10−3. (a) Initial state of the wave packet moving in the +xdirection. (b) After a time evolution of(Vhis the hopping energy for electrons), the wave packet is positioned just before the narrowest constriction in the QPC potential. (c) After a time evolution of, the wave packet is transmitted through the narrowest constriction. (d) Initial state of the wave packet moving in the −xdirection. (e) After a time evolution of. (f) After a time evolution of. Figure 2 shows the time evolution of the wave packet and the y direction spin density in the QPC channel calculated by the equation-of-motion method based on the exponential product formula [20] . Figure 2a shows the initial state of the electron wave packet moving in the + x direction without spin polarization. As the wave packet approaches the QPC potential, the down-spin (blue) wave packet moves to the centre of the channel, and the up-spin (red) wave packets then move to the top and the bottom of the channel ( Fig. 2b ). As the down-spin (blue) wave packet travels through the channel, the up-spin (red) wave packet is reflected by the QPC potential ( Fig. 2c ). As the effective magnetic field gradient d B eff /d y caused by the spatial modulation of the Rashba SOI generates a spin-dependent force F ↑↓ =± gμ B d B eff /d y , where g is the electron g -factor and μ B is the Bohr magneton, the spin-up and spin-down electron wave packets accelerate in opposite directions, resulting in a spin-dependent deflection as shown in Fig. 2b . This spin-separation mechanism is based on a non-uniform SOI, as was the theoretical proposal using the Stern–Gerlach spin filter [13] . The filtering function of the QPC demonstrated in this work can be attributed to the opposite spatial gradients of both sides of the lateral confinement potential along the y direction, which in effect induces a sign change of d B eff /d y . As a result, the down spin polarization is concentrated at the centre, where the potential energy for down spin is lower than that for up spin. This potential difference between up spin and down spin induces either a spin-dependent transmission or reflection at the QPC constriction depending on the electron spin ( Fig. 2c ). When the wave packet travels in the reverse (− x ) direction ( Fig. 2d–f ), the generated spin polarization shows the opposite sign due to the momentum-dependent effective magnetic field. Figure 2: Time evolution of the wave packet for the charge density and the spin density in the QPC channel. The three panels in a – f indicate the position of the electron wave packet, the charge density and the spin density in the QPC device. Colour bars beneath the panels correspond to scales of charge density between 0 and 2×10 −3 , and spin density between −2×10 −3 and +2×10 −3 . ( a ) Initial state of the wave packet moving in the + x direction. ( b ) After a time evolution of ( V h is the hopping energy for electrons), the wave packet is positioned just before the narrowest constriction in the QPC potential. ( c ) After a time evolution of , the wave packet is transmitted through the narrowest constriction. ( d ) Initial state of the wave packet moving in the − x direction. ( e ) After a time evolution of . ( f ) After a time evolution of . 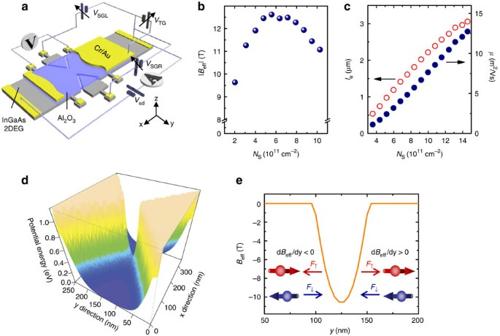Figure 3: Measurement setup and physical properties of the InGaAs-based QPC device. (a) The trench-type QPC device with top- and side-gate electrodes. The trench and surface of the device are covered with an Al2O3insulator. Although the top gate is not drawn around the QPC region for the clarity of the side gates, a Cr/Au top gate covers the entire QPC region in the real device. (b) Effective magnetic fieldBeffas a function of sheet carrier density in an InGaAsP/InGaAs two-dimensional electron gas atT=0.3 K. (c) Electron mean free path and mobility as a function of sheet carrier density in an InGaAsP/InGaAs two-dimensional electron gas atT=0.3 K. The red circles and blue circles are the electron mean free path and the mobility with the left and right axes, respectively. (d) Calculated potential landscape in an InGaAsP/InGaAs-based QPC. The potential structure is spatially modulated along the conducting channel due to the side gates. (e) Calculated effective magnetic fieldBeffalong the y direction atx=106 nm. Full size image Device structure and measurement setup Figure 3a shows our device and measurement configurations (also see device structure and fabrication in Methods). An InGaAsP/InGaAs heterostructure was designed to enhance the Rashba SOI and evaluated the Rashba SOI parameter α in a Hall bar device by measuring weak anti-localization at T =0.3 K (ref. 17 ). Rashba SOI parameter α is controlled between 5.3 and 10.4×10 −12 eVm by changing the top-gate bias voltage. The induced effective magnetic field is described by | B eff |=2| α | k F / gμ B , where k F is the Fermi wave number, g is the electron g -factor and μ B is the Bohr magneton. | g |=4.2 is evaluated from the Zeeman effect on the spin-dependent potential energy. Figure 3b shows the effective magnetic field as a function of sheet carrier density N S . The peak in the effective magnetic field is due to the opposite dependence of k F and α on N S. The maximum value of the effective magnetic field is higher than 12 T around N S =6×10 11 cm −2 . The carrier density dependence of the electron mean free path l e and mobility μ at T =0.3 K is shown in Fig. 3c . An epitaxial wafer was used for the fabrication of a trench-type QPC as shown in the scanning electron microscope image inset in Fig. 1 and a top-gate electrode was added. The side-gate voltage ( V SG ) controls the channel conductance, and the top-gate voltage ( V TG ) controls the carrier density and the strength of the Rashba SOI. We prepared three devices of different channel widths: 450 (device A), 400 (device B) and 360 nm (device C). Figure 3: Measurement setup and physical properties of the InGaAs-based QPC device. ( a ) The trench-type QPC device with top- and side-gate electrodes. The trench and surface of the device are covered with an Al 2 O 3 insulator. Although the top gate is not drawn around the QPC region for the clarity of the side gates, a Cr/Au top gate covers the entire QPC region in the real device. ( b ) Effective magnetic field B eff as a function of sheet carrier density in an InGaAsP/InGaAs two-dimensional electron gas at T =0.3 K. ( c ) Electron mean free path and mobility as a function of sheet carrier density in an InGaAsP/InGaAs two-dimensional electron gas at T =0.3 K. The red circles and blue circles are the electron mean free path and the mobility with the left and right axes, respectively. ( d ) Calculated potential landscape in an InGaAsP/InGaAs-based QPC. The potential structure is spatially modulated along the conducting channel due to the side gates. ( e ) Calculated effective magnetic field B eff along the y direction at x =106 nm. Full size image Figure 3d shows the calculated potential landscape in the present QPC. The application of voltage at the side gates results in carrier depletion in the channel and determines the energy potential gradient along the y direction. This induces the spatial modulation of the effective magnetic field ( Fig. 3e ). As the effective magnetic fields d B eff /d y exhibit opposite gradients at the sides of the QPC channel ( Fig. 3e ), a spin-dependent force concentrates one spin at the centre of the QPC ( Fig. 2b,e ). It should be noted that this is what distinguishes our experiment from the original Stern–Gerlach experiment [1] , [2] . Conductance measurement under an applied electric field We first measured conductance plateaus under different V TG in QPC device A and QPC device C to reveal the modulation effect of the effective magnetic field. Although V TG was fixed, V SG was swept to a negative bias with identical voltages between the left and right side gates ( V SGL and V SGR ). The red lines in Fig. 4a,b represent conductance ( G ) as a function of V SG for V TG =+5.8 and +1.7 V, respectively, at an external magnetic field B ex =0 T and temperature T =3.6 K. Clear conductance plateaus are observed from G =1(2 e 2 / h ) to 3(2 e 2 / h ) for QPC device A and G =5(2 e 2 / h ) for QPC device C in steps of 2 e 2 / h , indicating the formation of a one-dimensional channel by modulating the side gates. Recent shot-noise measurement unambiguously proves the quantized channel formation at these plateaus [21] . When V TG is reduced to +2.4 and +0.3 V, a half-integer plateau, shown by the blue lines in Fig. 4a,b , appears at 0.5(2 e 2 / h ), indicating the formation of a spin-polarized single channel. The decrease of V TG causes an increase in the Rashba SOI, indicating that the effective magnetic field B eff is responsible for the spin generation. 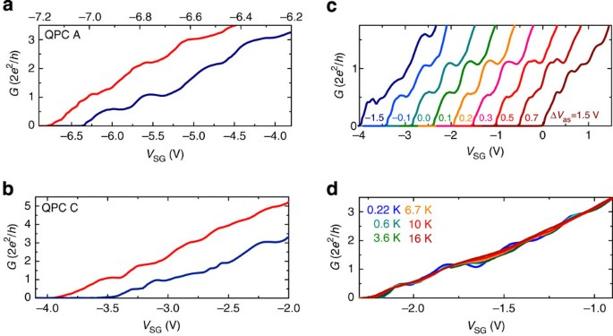Figure 4: Quantized conductance plateaus. The dependence of the QPC conductanceGon the side-gate voltageVSGfor different top-gate voltagesVTGwith different channel widths: 450 (device A) and 360 nm (device C). (a)VTG=+5.8 (red line) and +2.4 V (blue line) for QPC device A, and (b)VTG=+1.7 (red line) and +0.3 V (blue line) for QPC device C atBex=0 T andT=3.6 K. (c) AsymmetricVSGdependence onGatVTG=+2.4 V for QPC device A. The difference betweenVSGLandVSGRis defined asΔVas=VSGL−VSGR.ΔVasis kept constant during the sweeps ofVSGLandVSGR. (d) Temperature dependence of the conductance plateau atT=0.22–16 K atBex=0 T andVTG=+0.3 V for QPC device C. Figure 4: Quantized conductance plateaus. The dependence of the QPC conductance G on the side-gate voltage V SG for different top-gate voltages V TG with different channel widths: 450 (device A) and 360 nm (device C). ( a ) V TG =+5.8 (red line) and +2.4 V (blue line) for QPC device A, and ( b ) V TG =+1.7 (red line) and +0.3 V (blue line) for QPC device C at B ex =0 T and T =3.6 K. ( c ) Asymmetric V SG dependence on G at V TG =+2.4 V for QPC device A. The difference between V SGL and V SGR is defined as ΔV as = V SGL − V SGR . ΔV as is kept constant during the sweeps of V SGL and V SGR . ( d ) Temperature dependence of the conductance plateau at T =0.22–16 K at B ex =0 T and V TG =+0.3 V for QPC device C. Full size image To accurately determine the origin of the observed 0.5(2 e 2 / h ) plateau, and to be sure it was neither a lateral SOI [22] , [23] , [24] nor a 0.7(2 e 2 / h ) plateau [25] , [26] , we employed asymmetric side-gate bias and temperature dependences. The lateral SOI is induced by the asymmetric potential gradient along the lateral confinement direction ( y direction), which is modulated by the asymmetric bias between the left and right side gates in the QPC (for details, see Supplementary Discussion ). As the lateral SOI also acts as an effective magnetic field, it has been suggested that it may have a role in generating spin polarization [22] . The asymmetric side-gate bias dependence in QPC device A is shown in Fig. 4c for B ex =0 T and T =3.6 K. We applied different values of V SGL and V SGR under V TG =+2.4 V. During V SGL and V SGR sweeps, we maintained a constant voltage difference of ΔV as = V SGL − V SGR . Although the conductance plateaus at 0.5(2 e 2 / h ) and 1.0(2 e 2 / h ) were stable in −0.7 V≤ ΔV as ≤+0.7 V, further ΔV as (=±1.5 V) induces other plateaus in addition to 0.5(2 e 2 / h ) and 1.0(2 e 2 / h ). As the modulation of a lateral electric field by ΔV as does not have a role in the appearance or disappearance of 0.5(2 e 2 / h ), the lateral SOI can be ruled out as the origin of 0.5(2 e 2 / h ). Although a plateau-like structure around 0.7(2 e 2 / h ), the so-called 0.7 structure [25] , has been reported experimentally and theoretically [26] , the 0.5(2 e 2 / h ) plateau observed in this study becomes weaker at higher temperatures with the disappearance of integer plateaus ( Fig. 4d ). This does not occur in the 0.7 structure [25] , [26] , [27] . Rather, the 0.7(2 e 2 / h ) plateau remains even when the temperature increases. As the 0.5(2 e 2 / h ) behaves differently from the 0.7 structure [25] , [26] , [27] , it can be assumed to have another origin. Differential conductance analysis under an external magnetic field When the electron is approaching the QPC constriction, up spin and down spin are spatially separated by the spin-dependent force, F ↑↓ =± gμ B d B eff /d y , due to the spatial modulation of the effective magnetic field shown in Fig. 5a . This spatial separation of up spin and down spin corresponds to the formation of the spin-dependent potential along the y direction as depicted in Fig. 5b . For electrons moving in the + x direction, the potential energy for down spin at the channel centre is lower than that for up spin. This potential energy difference results in the concentration of down spin at the channel centre. 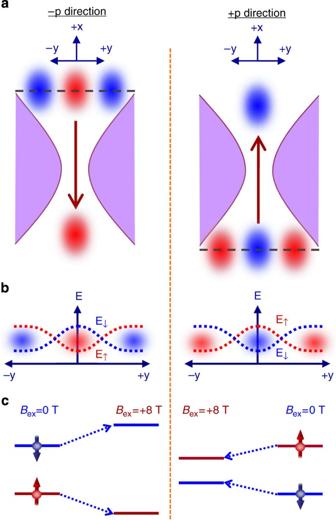Figure 5: Spin-dependent potential energy on opposite electron momentum directions and the effect of an external magnetic field. (a) Schematic model of the spin separation and transmission for positive (+p) and negative (−p) momentum directions. The red and blue ovals represent the spin-up and spin-down densities, respectively. (b) Corresponding spin-dependent potential energy along y direction at a black dashed lines inaindicated by the red and blue dashed lines for up spin and down spin, respectively. Opposite spin-dependent potential is induced at the channel centre of the QPC. (c) Schematic model of the spin-dependent potential energy and its evolution under the external magnetic fieldBex. The solid red and blue lines represent the energy levels between spin-up and spin-down potentials, respectively, at y=0. The spatial modulation of momentum-dependent effective magnetic field induces the spin-dependent potential energy with opposite spin direction in positive (+p) and negative (−p) momentum directions. The Hamiltonian of the SOI under the external magnetic field is described by Figure 5: Spin-dependent potential energy on opposite electron momentum directions and the effect of an external magnetic field. ( a ) Schematic model of the spin separation and transmission for positive (+p) and negative (−p) momentum directions. The red and blue ovals represent the spin-up and spin-down densities, respectively. ( b ) Corresponding spin-dependent potential energy along y direction at a black dashed lines in a indicated by the red and blue dashed lines for up spin and down spin, respectively. Opposite spin-dependent potential is induced at the channel centre of the QPC. ( c ) Schematic model of the spin-dependent potential energy and its evolution under the external magnetic field B ex . The solid red and blue lines represent the energy levels between spin-up and spin-down potentials, respectively, at y=0. The spatial modulation of momentum-dependent effective magnetic field induces the spin-dependent potential energy with opposite spin direction in positive (+p) and negative (−p) momentum directions. Full size image where is the intrinsic SOI parameter, σ is the Pauli-spin matrices, p is the electron momentum and E is the internal electric field along the z direction, which corresponds to the potential gradient of the quantum well, B eff is the effective magnetic field induced by the SOI, g is the electron g -factor, μ B is the Bohr magneton and B ex is the external magnetic field. It is noted that the sign of the effective magnetic field B eff depends on the electron momentum direction. The spin accumulation at the channel centre is opposite to the electron momentum direction, as described in Fig. 5b . The induced potential energy difference between up spin and down spin modulates the transmission probability for electrons to pass through the QPC constriction, resulting in the observation of a spin-resolved single channel as G =0.5(2 e 2 / h ) at B ex =0 T. As shown in Fig. 5c , when the external magnetic field is applied, the additional Zeeman energy either enhances or reduces this spin-dependent potential energy gap at the channel centre, depending on the electron momentum direction. As a result, the combination of the momentum-dependent effective magnetic field B eff and the external magnetic field B ex induces the asymmetric splitting of the spin-dependent potential energy. To confirm that the origin of the spin polarization is the SOI, we applied an external magnetic field B ex along B eff , achieving asymmetric spin splitting as expected in ± V sd ; |− E s + gμ B B ex | for + V sd and |+ E s + gμ B B ex | for − V sd , where E s and gμ B B ex are the spin-dependent potential energy gap at 0.5(2 e 2 / h ) and Zeeman energy, respectively. The differential conductance d G /d V SG measured in the QPC device C as functions of V sd and V SG at T =0.22 K under B ex =0 and +8 T (// B eff ) are shown in Fig. 6a,b . The black (low d G /d V SG. ) and red/yellow (high d G /d V SG. ) regions correspond to conductance plateaus and energy crossings between the top of the spin-dependent potential and the source and drain chemical potentials, respectively. At B ex =0 T, the energy crossing is almost symmetric to the ± V sd directions. The two red lines originating from V SG =−2.25 and −2.45 V cross each other around V sd =±5 mV corresponding to the simultaneous energy crossing of both source and drain chemical potentials, with adjacent spin-dependent potential energies. From the applied e V sd , we determine the spin-dependent potential energy gap: E s =5.05 meV for +V sd and 6.02 meV for −V sd . Our results indicate a larger energy difference between up spin and down spin than the values previously reported [22] , [28] , [29] , [30] . When we apply B ex =+8 T, the spin-dependent potential energy changes, becoming asymmetric in the ± V sd directions (see the dotted lines in Fig. 6b ). As the positive B ex is parallel (antiparallel) to the direction of the electron spins polarized by the spin-dependent potential in − V sd (+ V sd ), gμ B B ex is additive (subtractive) to E s , resulting in the further energy difference between up-spin and down-spin potentials in ± V sd . This asymmetric behaviour unambiguously proves that the observed 0.5(2 e 2 / h ) originates from momentum-dependent spin polarization. 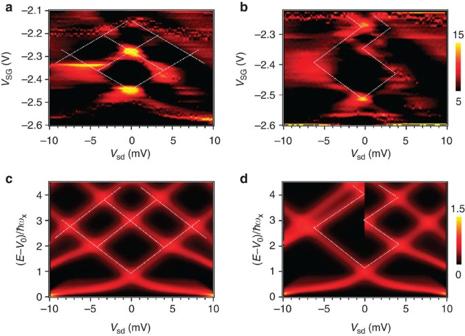Figure 6: Energy spectroscopy on spin-dependent potential as a function of source-drain bias voltage with/without an external magnetic field. The dotted white lines are traces of the energy crossings between the spin-dependent potential energy and the source/drain chemical potentials. The colour scales on the right indicate the differential conductance: 5 to 15 (ΩV)−1for the experiment and 0 to 1.5 (ΩV)−1for calculations. (a) Differential conductance dG/dVSGas functions ofVsdandVSGatBex=0 T andT=0.22 K. (b) dG/dVSGas functions ofVsdandVSGatBex=+8 T andT=0.22 K. (c) Calculated differential conductance as functions ofVsdand normalized electron energyatBex=0 T. (d) Calculated differential conductance as functions ofVsdand normalized electron energy atBex=+8 T. Figure 6: Energy spectroscopy on spin-dependent potential as a function of source-drain bias voltage with/without an external magnetic field. The dotted white lines are traces of the energy crossings between the spin-dependent potential energy and the source/drain chemical potentials. The colour scales on the right indicate the differential conductance: 5 to 15 (ΩV) −1 for the experiment and 0 to 1.5 (ΩV) −1 for calculations. ( a ) Differential conductance d G/ d V SG as functions of V sd and V SG at B ex =0 T and T =0.22 K. ( b ) d G/ d V SG as functions of V sd and V SG at B ex =+8 T and T =0.22 K. ( c ) Calculated differential conductance as functions of V sd and normalized electron energy at B ex =0 T. ( d ) Calculated differential conductance as functions of V sd and normalized electron energy at B ex =+8 T. Full size image To further confirm the relevance of the Rashba SOI, a differential conductance was calculated as a function of V sd and electron energy [31] (for a detailed calculation, see Supplementary Methods ). We considered the saddle-point potential and additional energy terms in an electron-transmission probability T n for each subband n; Zeeman energy ±1/2 gμ B B ex and momentum-dependent potential energy difference for up and down spins for −(+) V sd . Figure 6c,d shows the calculated results at B ex =0 and +8 T, respectively. The vertical axis represents the normalized electron energy ( E − V 0 / h ω x corresponding to the V SG , where E is the electron energy, V 0 is the bottom of the saddle-point potential and ω x describes the curvature of the inverted parabolic potential in the QPC. Symmetric potential energy evolution is reproduced at B ex =0 T. It is noted that the spin-dependent potential energy gap is equal but has opposite signs for ± V sd . As a result, the spin-polarized direction can be reversed by switching the V sd bias direction. At B ex =+8 T, the potential energy evolution becomes asymmetric to ± V sd because the potential energy difference for up and down spins shows for + V sd and ±1/2 E s ±1/2 gμ B B ex for − V sd . These characteristic features obtained in the calculation well reproduce our experimental observations by introducing for the −(+) V sd direction, indicating that the opposite spin-dependent potential energy for the electron momentum directions due to Rashba SOI has an essential role for generating 0.5(2 e 2 / h ). Shot-noise measurement For a quantitative evaluation of spin polarization at 0.5(2 e 2 / h ), we employed shot-noise measurement [29] , [30] in the QPC device B at B ex =0 T and T =4.2 K. Although conductance measurements only provide an average of the transmissions between the spin-up and spin-down channels, that is, , where τ σ are spin-up ( σ =↑) and spin-down ( σ =↓) transmissions, it has been shown that shot-noise measurements provide decomposed spin-dependent transmissions in the conducting channel [29] , [30] . When the dc current I is applied to the QPC, the shot noise yields the current fluctuation S I =2 eIF in the zero-temperature and zero-frequency limit, where the dimensionless parameter F is called the Fano factor to characterize the channel-dependent transmission process of electrons. The mesoscopic scattering theory predicts for G ≤ G 0 =(2 e 2 / h ), and F =1− G / G 0 when the spin is degenerated. However, owing to the asymmetric contribution of the two spin-dependent channels, the Fano factor is less than its theoretical value. As shown in Fig. 7a , the Fano factor around 0.5(2 e 2 / h ) is less than its theoretical zero spin polarization (the dashed-blue line) and is close to the full spin polarization (the dotted-red line). As the Fano factor is described by , we can extract τ ↑ and τ ↓ as a function of V SG (the red and blue circles in Fig. 7b ). The different values of the obtained τ ↑ and τ ↓ around 0.5(2 e 2 / h ) are clear evidence of the asymmetric contribution of the two spin-dependent channels to the conductance. The spin polarization defined by is shown in Fig. 7c . As V SG increases, P S decreases and gradually approaches zero when the conductance exceeds 0.5(2 e 2 / h ). At the 0.5(2 e 2 / h ) plateau, the maximum value reached is P S =0.7. It should be noted that this value of spin polarization is much higher than that of conventional Fe, Co and Ni ferromagnets ( P S ~ 0.4 to 0.5). 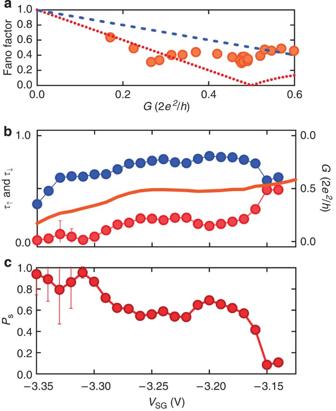Figure 7: Shot-noise measurement and spin polarization. (a) Fano factor as a function of the conductance,G. The dashed blue line shows the theoretical curve of zero spin polarization,F= 1 -G/G0(G0=2e2/h), and the dotted red line shows the case of full spin polarization. (b)VSGdependence of the conductanceGand the transmissionτσof up-spin (σ=↑) and down-spin (σ=↓) channels.τσis extracted from the measured conductanceand Fano factor. The fine lines through the circles indicate the degree of error. (c) Spin polarizationPSdefined byas a function ofVSG. At 0.5(2e2/h), the maximum value reachesPS=0.7. The error bars in panelbandcrepresent the standard deviation deduced from the numerical fitting procedure as a result of the experimental uncertainty of the Fano factor. Figure 7: Shot-noise measurement and spin polarization. ( a ) Fano factor as a function of the conductance, G . The dashed blue line shows the theoretical curve of zero spin polarization, F = 1 - G / G 0 ( G 0 =2 e 2 /h ), and the dotted red line shows the case of full spin polarization. ( b ) V SG dependence of the conductance G and the transmission τ σ of up-spin ( σ = ↑ ) and down-spin ( σ = ↓ ) channels. τ σ is extracted from the measured conductance and Fano factor . The fine lines through the circles indicate the degree of error. ( c ) Spin polarization P S defined by as a function of V SG . At 0.5(2 e 2 / h ), the maximum value reaches P S =0.7. The error bars in panel b and c represent the standard deviation deduced from the numerical fitting procedure as a result of the experimental uncertainty of the Fano factor. Full size image The spin-separation angle γ SGE is described by where l e is the mean free path, E F is 1/2 m * v 2 F and E eff is gμ B B eff . The estimated γ SGE under V TG =0.3 V in the QPC device C is 0.65 after taking the mean free path ( l e =2.4 μm), the carrier density ( N S =1.27×10 12 cm −2 ), the Rashba SOI parameter (3.74×10 −12 eVm) and the effect of carrier depletion in the QPC into consideration. This value is much larger than spin Hall angles γ SHE obtained experimentally till date [10] , suggesting that the utilization of the spatially modulated Rashba SOI for spin separation is more efficient. The theoretical calculations shown in Fig. 2 reflect our expectation that the generated spin polarization would have opposite signs in the positive and negative moving direction for electron due to the momentum-dependent effective magnetic field. In fact, our experimental findings, shown in in Fig. 6 , confirm this characteristic feature. The opposite spin-dependent potential between positive and negative source-drain bias directions was confirmed by applying an external magnetic field parallel to the effective magnetic field direction, and is clear evidence that the spin separation is due to the Rashba SOI. The spin-dependent force due to the spatial modulation of the effective magnetic field concentrates either down or up spins at the centre of the QPC channel depending on the momentum direction ( Fig 2b,e ), resulting in a potential energy difference for up spin and down spin. This provides the asymmetric transmission probability between spin-up and spin-down electrons in the QPC. The quantum shot-noise measurements in Fig. 7b clearly indicate the spin-dependent transmission and are evidence that we successfully separated electron spin, not by using an external field as was the case in the Stern–Gerlach experiment, but by utilizing the spatial modulation of Rashba SOI in the InGaAs-based QPC structure. The spatially modulated SOI induced spin separation, and the QPC potential selectively filtered the spin of the conduction electrons. The obtained conductance plateau was a spin-resolved half integer with a unit value of 2 e 2 / h . With polarization as high as 70% of the conduction electrons, this technique has potential for application in semiconductor-based spintronic devices. The spin-separation technique used in the InGaAs-based QPC explained in this paper is simple and robust, and allows efficient spin generation and detection in semiconductor nanostructures without the need for magnetic fields or magnetic materials and, as such, paves the way towards the integration of electrical spin generation, manipulation and detection in future semiconductor-based spintronic devices and quantum information technology. Device structure and fabrication The sample was epitaxially grown on a (001) InP substrate by metal organic chemical vapour deposition. It consisted of the following—from the top: 25-nm In 0.52 Al 0.48 As; 3-nm (In 0.52 Al 0.48 As) 0.3 (In 0.53 Ga 0.47 As) 0.7 ; 10-nm In 0.8 Ga 0.2 As for a quantum well; 5-nm (In 0.53 Ga 0.47 As) 0.41 (InP) 0.59 ; 15-nm In 0.52 Al 0.48 As for a spacer layer; 6-nm In 0.52 Al 0.48 As for a carrier supply (Si doping with N d =4×10 18 cm −3 ); and 200-nm In 0.52 Al 0.48 As for a buffer layer. We designed the heterostructure such that a high electron probability density was positioned near the (In 0.53 Ga 0.47 As) 0.41 (InP) 0.59 /In 0.8 Ga 0.2 As interface to enhance the interface contribution of Rashba SOI [17] . QPCs were fabricated by electron beam lithography and reactive ion-etching techniques. The QPC was designed to have a width ( W ) of 300≤ W ≤500 nm. To improve side-gate controllability by filling trenches and provide a top-gate insulator, 150 nm Al 2 O 3 was formed by an atomic layer deposition. To form a top-gate electrode, 5-nm Cr/150-nm Au was evaporated and lifted off. AuGeNi (200 nm) was evaporated for voltage probes and source-drain electrodes, and annealed at 275 °C for 7 min for ohmic contact. Four-terminal measurements were performed by applying the source-drain voltage to probe the quantized conductance as functions of the gate voltages and external magnetic fields. The external magnetic field was applied parallel to the effective magnetic field for differential conductance measurements. We measured the carrier density and mobility in the Hall bar device connected to the QPC in series. We independently measured the basic properties of the two-dimensional electron gas in a gate-fitted Hall bar with a channel 20 μm in width and 80 μm in length. How to cite this article: Kohda, M. et al . Spin–orbit induced electronic spin separation in semiconductor nanostructures. Nat. Commun. 3:1082 doi: 10.1038/ncomms2080 (2012).